A new sauropod dinosaur from the Early Cretaceous of Tunisia with extreme avian-like pneumatization Recent interpretations of the postcranial anatomy of sauropod dinosaurs differ about pneumatic features supporting an avian-like ventilatory system; the most conservative workers reject most postcranial pneumatizations as being unambiguous evidence of abdominal air sacs. Here we describe the first articulated dinosaur skeleton from Tunisia and refer it to a new rebbachisaurid sauropod, Tataouinea hannibalis gen. et sp. nov. The Tunisian specimen shows a complex pattern of caudosacral and pelvic pneumatization—including the first report of an ischial pneumatic foramen among Dinosauria—strongly supporting the presence of abdominal air sacs. Character optimization among Rebbachisauridae indicates that in the caudal vertebrae, pneumatization of the neural arches preceded that of the centra; in the pelvis, pneumatization of the bones adjacent to the sacrum preceded that of more distal elements. Tataouinea was more closely related to European nigersaurines than to otherwise Gondwanan rebbachisaurids; this supports an Afro-European route for rebbachisaurid dispersal. Cretaceous dinosaurs of the peri-Mediterranean regions are the subject of an increasing number of studies focusing on some of the most important and debated topics in vertebrate palaeontology, inter alia Cretaceous biogeography and insular faunas, biodiversity, timing of radiation of groups and phylogenetic relationships among Gondwanan dinosaur clades with respect to their European counterparts [1] , [2] , [3] , [4] , [5] , [6] , [7] , [8] , [9] , [10] , [11] . In addition, Mediterranean dinosaur remains, particularly northern African specimens, are important for understanding some of the most extreme Cretaceous ecosystems. Diverse vertebrate faunas are known from calcareous platforms, islands and xeric coastal plains, often inhabited by endemic forms. Although the fossil record from these deposits consists mostly of incomplete specimens, diagnostic elements document unique characters interpreted as a reflection of special adaptations to exceptional combinations of ecological and climatic factors [2] , [7] , [12] , [13] , [14] . Field investigations in the Early Cretaceous deposits of the Tataouine region of southern Tunisia ( Fig. 1 ) in collaboration with the Office National Des Mines (ONM) in Tunis has led to discovery of the first articulated dinosaur skeleton from that country ( Fig. 2 ). The specimen, unfortunately, was seriously fissured during its transportation to Tunis. Detailed analysis indicate a complex pattern of caudosacral and pelvic pneumatization as well as the first report of an ischial pneumatocoel in a dinosaur, strongly supporting the presence of avian-like ventilatory air sacs extended posterior to the thoracic region. Available data allow us to refer this specimen to a new genus and species of rebbachisaurid sauropod, T. hannibalis . 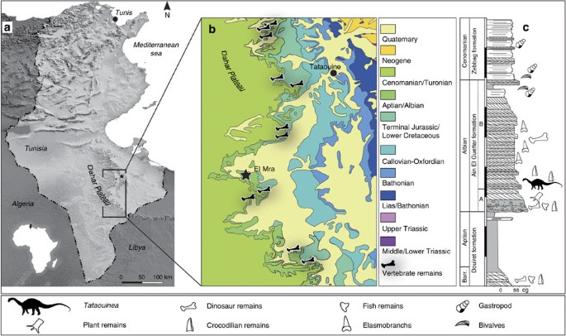Figure 1: Geological setting. (a) Reference map of the Tataouine region in southern Tunisia. (b) Geological map of the study area showing the distribution of Mesozoic deposits and the El Mra locality. (c) Stratigraphic field-log of the El Mra section. The Ain El Guettar Formation consists of the Chenini Member (a) and the Oum ed Diab Member (b).Tataouineawas collected from the basal beds of the early Albian Oum ed Diab Member. Figure 1: Geological setting. ( a ) Reference map of the Tataouine region in southern Tunisia. ( b ) Geological map of the study area showing the distribution of Mesozoic deposits and the El Mra locality. ( c ) Stratigraphic field-log of the El Mra section. The Ain El Guettar Formation consists of the Chenini Member ( a ) and the Oum ed Diab Member ( b ). Tataouinea was collected from the basal beds of the early Albian Oum ed Diab Member. 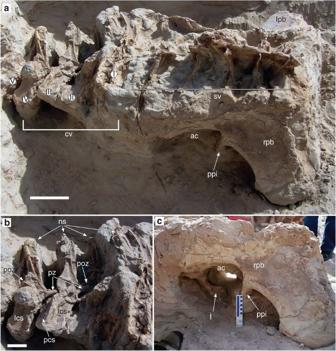Figure 2:T. hannibalisholotypein situ. (a–c) Field photographs of ONM DT 1–36 showing the articulation of elements. (a) Right dorsolateral view. (b) Detail of the caudal vertebrae in lateral view. (c) Detail of the right acetabular region in lateral view. I–V, caudal centra; ac, acetabulum; cv, caudal vertebrae; i, ischium; lcs, lateral centrum surface; lpb, left preacetabular blade; ns, neural spine; pcs, posterior centrum surface; poz, postzygapophysis; ppi, pubic peducle of ilium; pz, prezygapophysis; rpb, right preacetabular blade; sv, sacral vertebrae. Scale bar: 20 cm (a), 10 cm (b,c). Full size image Figure 2: T. hannibalis holotype in situ . ( a – c ) Field photographs of ONM DT 1–36 showing the articulation of elements. ( a ) Right dorsolateral view. ( b ) Detail of the caudal vertebrae in lateral view. ( c ) Detail of the right acetabular region in lateral view. I–V, caudal centra; ac, acetabulum; cv, caudal vertebrae; i, ischium; lcs, lateral centrum surface; lpb, left preacetabular blade; ns, neural spine; pcs, posterior centrum surface; poz, postzygapophysis; ppi, pubic peducle of ilium; pz, prezygapophysis; rpb, right preacetabular blade; sv, sacral vertebrae. Scale bar: 20 cm ( a ), 10 cm ( b , c ). Full size image Skeletal remains of Tataouinea were obtained from the Oum ed Diab Member of the Ain el Guettar Formation at the Jebel El Mra ( Fig. 1 ): these beds were dated as early Albian based on lateral correlation with marine units and associate vertebrate fauna [15] . Overall, the Oum ed Diab Member represents sandy shoreface (low angle to cross-bedded structures) and tidal flat/foreshore deposits (dominated by typical bidirectional tidal foreset and flaser stratification). Unidirectional, large cross-bedding structures indicate conditions of rapid deposition: the preservation of fully articulated pelvic and vertebral column elements are consistent with minor pre-burial transport of the carcass. Rare in situ plant roots are consistent with sparsely vegetated ground and relatively low water depth. Elasmobranchs, actinopterygians, sarcopterygians, crocodyliforms, pterosaurs and minor non-avian dinosaur elements (that is, spinosaurid, carcharodontosaurid and abelisaurid teeth) have been found at the El Mra locality. In particular, abundant crocodyliform remains referable to four clades (notosuchians, pholidosauroids, sebecids and eusuchians), and seven genera of sharks greatly outnumber all other vertebrate remains. These data, combined with a basin-scale facies analysis of the Oum ed Diab deposits [15] , indicate a vast mouth-bar environment characterized by both fluvial and tidal influence and dominated by marine taxa. Isolated, sauropod distal caudal vertebrae associated with large crocodilian teeth obtained about 20 metres from the main quarry may indicate scavenging of the carcass. Systematic palaeontology Dinosauria Owen, 1842 Saurischia Seeley, 1888 Sauropoda Marsh, 1878 Rebbachisauridae Bonaparte, 1997 Nigersaurinae Whitlock, 2011 Tataouinea hannibalis gen. et sp. nov Etymology. The genus name refers to the Tataouine Governatorate, Tunisia. The species name refers to Hannibal Barca (247-183 BC), Carthaginian military commander who marched an army including war elephants across Southern Europe. Holotype. ONM DT 1–36, sacrum, the five anteriormost caudal vertebrae, both ilia, both ischia ( Figs 2 , 3a–j and 4a–g ). Type locality and horizon. Ain el Guettar Formation, Oum ed Diab Member, Jebel El Mra, southern Tunisia; early Albian [15] . Estuarine to shallow marine deposits showing fining-upward sequences of fine-graded sandstones with herringbone cross-bedding, symmetrical wave-formed ripples and discontinuous clay lenses. Diagnosis. Large rebbachisaurid sauropod dinosaur with unique combination of completely fused sacral neural spines 1–3; camellate anterior sacral neural spines, semicamellate [16] posterior sacral neural spines; elliptical foramen in lateral surface of fourth sacral neural spine penetrating the camerate sector of the spine (autapomorphy); anteriormost caudal vertebrae with large elliptical pleurocoel in the lateral surface of centrum (autapomorphy); pneumatic foramen in the spinoprezygapophyseal fossa of anterior caudal vertebrae; pneumatic foramen in the prezygospinodiapophyseal fossa of anterior caudal vertebrae; ‘lateral lamina’ in anterior caudal neural spines is ‘inverted Y’-shaped, formed by the spinoprezygapophyseal and spinodiapophyseal laminae merging in the ventral third of spine and bordering a triangular fossa (autapomorphy); pubic peduncle of ilium hollowed by a large chamber; ischium with large elliptical foramen in the medial surface of the iliac peduncle (autapomorphy). 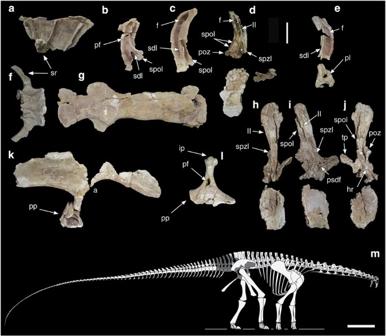Figure 3:T. hannibalisselected elements and reconstruction. (a) Sacral neural arches 1–3, right lateral view; (b) sacral neural spine 4, right lateral view; (c) sacral neural spine 5, right lateral view; (d) caudal vertebra 2 and fragment of caudal 1 postzygapophyses, left lateral view; (e) caudal vertebra 1, left lateral view; (f) sacral centrum 1, ventral view; (g) sacral centra 2–5, ventral view; (h–j) caudal vertebra 3, anterior (h), left lateral (i), posterior (j) views; (k) left ilium, lateral view; (l) right ischium, medial view; and (m) skeletal reconstruction ofT. hannibalis. Missing elements based on other nigersaurines. Scale bar: 10 cm (a–l), 1 m (m). a, acetabulum; f, fossa; hr, hyposphenal ridge; ip, ischial peduncle; ll, lateral lamina; pf, pneumatic foramen; pl, pleurocoel; poz, postzygapophysis; pp, pubic peduncle; psdf, prezygospinodiapophyseal foramen; sdl, spinodiapophyseal lamina; spol, spinopostzygapophyseal lamina; spzl, spinoprezygapophyseal lamina; sr, sacral rib; tp, transverse process. The asterisk indicates the fossa bounded by the spzl and the sdl. Figure 3: T. hannibalis selected elements and reconstruction. ( a ) Sacral neural arches 1–3, right lateral view; ( b ) sacral neural spine 4, right lateral view; ( c ) sacral neural spine 5, right lateral view; ( d ) caudal vertebra 2 and fragment of caudal 1 postzygapophyses, left lateral view; ( e ) caudal vertebra 1, left lateral view; ( f ) sacral centrum 1, ventral view; ( g ) sacral centra 2–5, ventral view; ( h – j ) caudal vertebra 3, anterior ( h ), left lateral ( i ), posterior ( j ) views; ( k ) left ilium, lateral view; ( l ) right ischium, medial view; and ( m ) skeletal reconstruction of T. hannibalis . Missing elements based on other nigersaurines. Scale bar: 10 cm ( a – l ), 1 m ( m ). a, acetabulum; f, fossa; hr, hyposphenal ridge; ip, ischial peduncle; ll, lateral lamina; pf, pneumatic foramen; pl, pleurocoel; poz, postzygapophysis; pp, pubic peduncle; psdf, prezygospinodiapophyseal foramen; sdl, spinodiapophyseal lamina; spol, spinopostzygapophyseal lamina; spzl, spinoprezygapophyseal lamina; sr, sacral rib; tp, transverse process. The asterisk indicates the fossa bounded by the spzl and the sdl. 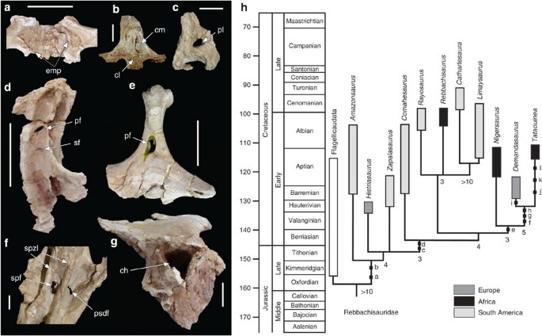Figure 4: Pneumatic features ofT. hannibalis. (a–g) Selected elements ofT. hannibalisshowing osteological correlates of pneumatic features. (a) Partial sacral centrum, internal view; (b) fourth sacral neural spine, transverse section; (c) anterior caudal centrum, lateral view; (d) fourth sacral neural spine, lateral view; (e) right ischium, medial view; (f) anterior caudal neural arch, detail in anterodorsal view; (g) pubic peduncle of ilium, cross-section. Scale bar: 10 cm (a,d,e); 5 cm (c,g); 2 cm (b,g). (h) Stratigraphically calibrated cladogram showing rebbachisaurid affinities ofTataouinea(relationships among non-rebbachisaurid taxa were omitted for brevity). Numbers adjacent to nodes indicate Decay Index values. Letters along branches indicate osteological correlates of pneumatic features21,26,39optimized under accelerated transformation: a, expansion of the pleurocoel in the dorsal surface of parapophysis in middle and posterior cervical centra; b, small chambers in the iliac blades; c, caudal centra with shallow lateral fossae; d, deep centroprezygapophyseal fossae in anterior caudal vertebrae; e, large pneumatic fossae between the spinodiapophyseal and the spinopostzygapophyseal fossae in the caudal vertebrae; f, semicamellate sacral neural spines; g, foramen in sacral neural spine; h, hollow pubic peduncle of ilium; i, ventral hollow in anterior caudal centra; j, triangular fossa in neural spines of anterior caudals; k, pleurocoelic caudal centra; and l, ischial pneumatization. ch, chamber; cl, camellae; cm, camerae; emp, extramural pneumatization; pf, pneumatic foramen; pl, pleurocoel; psdf, prezygospinodiapophyseal foramen; sf, semilunate fossa; spf, spinoprezygapophyseal foramen; spzl, spinoprezygapophyseal lamina. Full size image Figure 4: Pneumatic features of T. hannibalis . ( a – g ) Selected elements of T. hannibalis showing osteological correlates of pneumatic features. ( a ) Partial sacral centrum, internal view; ( b ) fourth sacral neural spine, transverse section; ( c ) anterior caudal centrum, lateral view; ( d ) fourth sacral neural spine, lateral view; ( e ) right ischium, medial view; ( f ) anterior caudal neural arch, detail in anterodorsal view; ( g ) pubic peduncle of ilium, cross-section. Scale bar: 10 cm ( a , d , e ); 5 cm ( c , g ); 2 cm ( b , g ). ( h ) Stratigraphically calibrated cladogram showing rebbachisaurid affinities of Tataouinea (relationships among non-rebbachisaurid taxa were omitted for brevity). Numbers adjacent to nodes indicate Decay Index values. Letters along branches indicate osteological correlates of pneumatic features [21] , [26] , [39] optimized under accelerated transformation: a, expansion of the pleurocoel in the dorsal surface of parapophysis in middle and posterior cervical centra; b, small chambers in the iliac blades; c, caudal centra with shallow lateral fossae; d, deep centroprezygapophyseal fossae in anterior caudal vertebrae; e, large pneumatic fossae between the spinodiapophyseal and the spinopostzygapophyseal fossae in the caudal vertebrae; f, semicamellate sacral neural spines; g, foramen in sacral neural spine; h, hollow pubic peduncle of ilium; i, ventral hollow in anterior caudal centra; j, triangular fossa in neural spines of anterior caudals; k, pleurocoelic caudal centra; and l, ischial pneumatization. ch, chamber; cl, camellae; cm, camerae; emp, extramural pneumatization; pf, pneumatic foramen; pl, pleurocoel; psdf, prezygospinodiapophyseal foramen; sf, semilunate fossa; spf, spinoprezygapophyseal foramen; spzl, spinoprezygapophyseal lamina. Full size image Description The firmly, co-ossified sacral centra show barely visible intercentral sutures. The sacral centra exhibit extensive extramural pneumatization [17] . The anterior sacral neural arches are firmly co-ossified together, with the neural spines 1–3 forming a narrow and continuous sheet of bone resulting from coalescence of the pre- and postspinal laminae. In the sacrum, both spinodiapophyseal and spinozygapophyseal laminae are prominent. The three anteriormost sacral neural spines show a camellate internal structure and relatively simple external lamination, as in titanosauriforms [16] . The posteriormost two sacral neural spines show semicamellate internal structure [16] , deep and elliptical lateral fossae, and a prominent spinodiapophyseal lamina. The fourth sacral neural spine bears a small elliptical foramen in the lateral surface, anterior to the spinodiapophyseal lamina. The spinal foramen shows clearly defined margins and is present symmetrically in both sides of the lateral surface, leading to the corresponding camerate sector of the semicamellate structure. A semilunate fossa is present ventral to the left foramen; it likely represents incipient pneumatization [18] . The first five caudal vertebrae were preserved in their anatomical series ( Fig. 2a ). The caudal vertebrae show anteroposteriorly compressed procoelous centra taller than long, and neural spinae about 150% taller than centrum height. Large elliptical pleurocoels open on the lateral surface of the anteriormost caudal centra. The boss-like eminence anteroventral to the prezygapophyses as in European Nigersaurinae is absent [19] , [20] . In anterior view, the neural spines are ‘petal-shaped’, as in most diplodocoids [21] . Both pre- and postspinal laminae are present and mediolaterally prominent, and border deep elliptical fossae. It is unclear whether the lateral triangular processes, as seen in the caudal neural spines of other Nigersaurinae [19] , were present. The spinoprezygapophyseal laminae are prominent. In their anteroventral third, the spinoprezygapophyseal laminae are thickened, boss-like, and border a deep and narrow elliptical fossa housing a large foramen that enters a small chamber. An elliptical foramen opens in both the prezygospinodiapophyseal fossae [22] . The spinodiapophyseal lamina is prominent, and joins the spinoprezygapophyseal lamina at about 1/3 of spine height, forming a vertically directed ‘lateral lamina’. The joined spinoprezygapophyseal and spinodiapophyseal laminae enclose a triangular fossa, here interpreted as autapomorphic for T. hannibalis . The spinoprezygapophyseal lamina fails to contact the spinopostzygapophyseal lamina, differing from the Limaysaurinae [19] . The postspinal lamina does not expand mediolaterally as in other Nigersaurinae [19] . The dorsal surface of the left postzygapophysis in the fourth caudal shows a ‘hinge-like’ structure formed by a series of transversely oriented indentations. Given its absence in the right postzygapophysis, the feature is considered an abnormality. A robust hyposphenal ridge is present ventral to the postzygapophyses, as in Demandasaurus . All neural spines are posterodorsally directed, with the anteriormost scimitar-shaped (as in Cathartesaura and Zapalasaurus [23] ) and the posterior straight (as in Limaysaurus and Nigersaurus [13] , [24] ). The anterior half of both ilia were found in articulation with the sacrum. The preacetabular blade of ilium is a bluntly rounded trapezoid, similar to Amazonsaurus [25] , and hollowed by moderately sized chambers, as reported in a few other sauropods [26] . The slender pubic peduncle is subtriangular in cross-section and hollowed by a large chamber. The proximal half of both ischia are preserved. Each ischium was found articulated with the corresponding ilium ( Fig. 2c ). The acetabular margin of the ischium is constricted in the middle. The iliac peduncle of ischium bears a distinct neck. In the medial surface, at the level of the contact between the iliac and the pubic peduncles, a large elliptical foramen is present. The foramen shows clearly defined margins; it displays no evidence of being a preservational artefact. The main axis of the foramen is subequal to minimum width of the iliac peduncle, and is aligned with the main axis of the latter. In the left ischium, the collapse of the medial surface of the iliac peduncle indicates the presence of an internal chamber. The inner chamber opened by the medial foramen is roofed laterally by a narrow lamina. The laterodorsal margin of the ischium bears a prominent rugosity. The Tunisian sauropod includes the most complete sacrum of a rebbachisaurid known, providing important information on the morphology and phylogenetic affinities of this clade. Although a precise quantification of total body size of ONM DT 1–36 is not possible, comparison between its sacrum and the sacra of more complete diplodocoid specimens suggests an individual at least 14 m long [27] ( Table 1 ), thus more than 150% the adult length of Nigersaurus [13] . The holotype of T. hannibalis is interpreted to represent an ontogenetically mature individual based on the combination of large size, co-ossification of the sacrum, obliterated neurocentral suture in caudal vertebrae ( Fig. 2b ), and extensive pneumatization of the pelvic and caudal region [18] . Table 1 Sacrum and total body lengths of selected diplodocoids. Full size table Tataouinea shows a complex pattern of caudosacral and pelvic pneumatization, including (1) caudal pleurocoels leading to camerae, the first report in Rebbachisauridae; (2) sacral neural spines with foramina leading to a semicamellate internal structure, the first report in Diplodocoidea [16] ; (3) a large pneumatic chamber in the pubic peduncle of ilium, the first report in Sauropoda [26] ; and (4) ischial pneumatization, the first report in Dinosauria. The large, elliptical foramen in the medial surface of the ischium of Tataouinea does not differ in shape, depth and presence of clearly defined margins, from the pleurocoels in the axial skeleton and is interpreted as pneumatic in origin. Pneumatic invasion of the pelvic girdle has been reported in both theropods and neosauropods [18] , [26] , [28] , but all previous reports were limited to the ilium. Other sauropods show small internal chambers pneumatising the iliac blades but not invading the pubic peduncle [26] , whereas a large chamber hollowing the latter peduncle was reported only in theropods [28] . The distribution of the osteological correlates of pneumatic features among Rebbachisauridae shows a progressive expansion of the postcranial pneumatization along the lineage leading to nigersaurines ( Fig. 4b ). Character optimization indicates that in the caudal vertebrae, neural arch pneumatization preceded the pneumatization of the centra, a pattern also reported in theropods [29] (neural arch-first) and thus synapomorphic for Saurischia. In the pelvis, pneumatization of the iliac blades, bones adjacent to the axial skeleton, preceded the pneumatization of the pubic peduncle of ilium and the ischium, bones not in direct vertebral contact, following a ‘proximal-first patter’. Large pneumatopores penetrating the caudosacral vertebrae were considered as indication of abdominal air sacs [29] , [30] , a necessary component of the avian-like lung ventilation system [18] . A more conservative approach [28] considered axial pneumatization as ambiguous evidence of abdominal air sacs, and only pelvic pneumatization in areas removed from contact with the sacrum as unambiguous evidence of abdominal air sacs, to avoid potential confusion with extramural pneumatization by posterior expansions of the cervical air sacs. ONM DT 1–36 is the first sauropod where large pneumatic foramina penetrate pelvic bones removed from direct contact with the axial skeleton, and thus accords with the presence of abdominal air sacs even following the most conservative approach [28] . The Cretaceous vertebrate faunas of northern Africa are of considerable importance in terms of paleobiogeography, palaeoecology and evolution. On one side, mid-Cretaceous paralic ecosystems of the peri-Mediterranean area are represented by a rich and diversified fauna indicative of extremely productive biota with significant peaks in biodiversity observed in shallow marine and brackish taxa (including crocodilians) [15] , [31] , [32] . At the same time, some of the largest known terrestrial vertebrates, and in particular theropod and sauropod dinosaurs, have been found at the very margin of these ecosystems in an increasing number of localities [2] , [9] , [33] , [34] , [35] , [36] , [37] supporting adaptation of terrestrial taxa to extreme, xeric and poorly vegetated environments. Even though the abundance of both fishes and crocodilians may have represented a continual source of food for predatory theropods [38] , the presence of large-bodied herbivores such as Tataouinea in under-vegetated areas is puzzling. Tataouinea shows closest affinities with the Iberian Demandasaurus than with other African [13] or South American taxa [23] , [24] , [25] . Accordingly, a European lineage of nigersaurines results bracketed by North African taxa; the latter clade is part of a mainly Gondwanan radiation. Although complicated by the basal phylogenetic position of Histriasaurus from Croatia [34] , the resulted phylogenetic framework supports the hypothesis that rebbachisaurids originated in Gondwana before its fragmentation and reached Europe across the Tethyan carbonate platforms [20] , [34] . Phylogenetic analysis In order to establish the phylogenetic affinities of Tataouinea , we entered an Operational Taxonomic Unit based on ONM DT 1–36 in a recent phylogenetic analysis of Sauropoda [39] . The analysis recovered 12 shortest trees of 1,013 steps each (Consistency Index=0.3988, Retention Index=0.7251; Fig. 3H ). Tataouinea resulted among nigersaurine rebbachisaurids, closer to Demandasaurus than to Nigersaurus , based on the combination of hyposphenal ridge in caudal neural arches, elliptical fossae bordered by the ‘lateral’ and the spinopostzygapophyseal laminae in caudal neural spines, and iliac peduncle of ischium with distinct neck. Character scores of T. hannibalis Character states of the operational taxonomic unit based on ONM DT 1–36 entered in the phylogenetic analysis of Carballido et al. (2012) [39] and supporting the placement of Tataouinea among rebbachisaurids: ? ????????????????????????????????????????????????????????????????????????? ??????????????????????????????????????????????????????????????????????????? ???????????????????????????????211??1?1?0014100?0110?1?101?0???????????????????????????????? ?????????????????????????????????????11?01?????111?1?11?1??????????????????????????????????????????? (ref. 39 ) Osteological correlates of pelvic pneumatization The preacetabular blade of ilium is hollowed by small internal chambers [26] . The pubic peduncle of the ilium bears an internal chamber [16] , the latter occupying most of the volume [40] , [41] . Based on the cross-section area of the pubic peduncle, the peduncle has an air-space proportion value [17] of 0.65, in the upper range of values known in the diaphyses of pneumatised long bones in extant birds (0.59–0.64 ref. 17 ). Also, the inner side of the peduncle cortical bone bears a series of horizontal septa (about 10 mm thick), the latter defining a camerate pattern [16] . In the ischium, a large opening is present in the medial surface of iliac peduncle, being it one order of magnitude the size of neurovascular openings [42] . This opening is of regular shape and shows distinct margins [42] . The ischial foramen is extremely similar in shape and proportions to the pleurocoels in the caudal vertebrae: both are ellipses, with eccentricity of 0.87 and 0.93, respectively. The foramen leads to an internal chamber [17] , [29] . Nomenclatural acts This published work and the nomenclatural acts it contains have been registered in ZooBank, the proposed online registration system for the International Code of Zoological Nomenclature (ICZN). The ZooBank LSIDs (Life Science Identifiers) can be resolved and the associated information viewed through any standard web browser by appending the LSID to the prefix ‘ http://zoobank.org/ ’. The LSIDs for this publication are urn:lsid:zoobank.org:act:64D4BEAE-0941-4964-A889-EE5133852116 ( Tataouinea ) and urn:lsid:zoobank.org:act:7A7AD9CA-4051-4100-9E70-D94D12C8F093 ( T. hannibalis ). How to cite this article: Fanti, F. et al. A new sauropod dinosaur from the Early Cretaceous of Tunisia with extreme avian-like pneumatization. Nat. Commun. 4:2080 doi: 10.1038/ncomms3080 (2013).